Near-field interferometry of a free-falling nanoparticle from a point-like source Matter-wave interferometry performed with massive objects elucidates their wave nature and thus tests the quantum superposition principle at large scales. Whereas standard quantum theory places no limit on particle size, alternative, yet untested theories—conceived to explain the apparent quantum to classical transition—forbid macroscopic superpositions. Here we propose an interferometer with a levitated, optically cooled and then free-falling silicon nanoparticle in the mass range of one million atomic mass units, delocalized over >150 nm. The scheme employs the near-field Talbot effect with a single standing-wave laser pulse as a phase grating. Our analysis, which accounts for all relevant sources of decoherence, indicates that this is a viable route towards macroscopic high-mass superpositions using available technology. Matter-wave interference with particles of increasing size and mass is a natural and viable method for testing the validity of the quantum superposition principle at unprecedented macroscopic scales [1] , [2] , [3] , [4] . Macroscopic path separations are nowadays routinely achieved in atom interferometry [5] , [6] , [7] , and technological advances in the control of opto-mechanical systems [8] promise that much more massive objects may be delocalized [9] , [10] , [11] , [12] , [13] , albeit with spatial separations smaller than a single atom. Recent proposals put forward nanoparticle interferometry [14] , [15] in the mass range of 10 6 –10 9 AMU to surpass the mass records currently held by molecule diffraction experiments [3] , [16] , while maintaining spatial separations large enough to be resolved by optical means. A first demonstration with molecular clusters [15] is still far away from the mentioned high-mass regime due to difficult experimental challenges, mainly concerning the source and detection. The realization of a proposed double-slit scheme with silica nanospheres [14] requires motional ground-state cooling, which is an equally challenging task. Quite recently, optical feedback cooling has been demonstrated for 100-nm-sized particles [17] , [18] , based on pioneering work that demonstrated the trapping of polystyrene and glass microspheres [19] , trapping of viruses and bacteria [20] and even of complete cells [21] in solutions and high vacuum. Cavity cooling of particles of similar size was proposed [22] and recently achieved [23] , [24] in one dimension, with temperatures in the milli-Kelvin range. Although this is still far above the ground state of a typical 100-kHz trap, we will argue that high-mass interference can be realized experimentally with motional temperatures already achieved by optical cooling. In this paper, we present a near-field interference scheme for 10 6 AMU particles. It is based on the single-source Talbot effect [25] due to a single optical phase grating, as opposed to the three-grating scenario in Talbot–Lau interference experiments [3] . Optically trapped silicon nanospheres, feedback-stabilized to a thermal state of about 20 mK, provide a sufficiently coherent source. Individual particles are dropped and diffracted by a standing UV laser wave, such that interference of neighbouring diffraction orders produces a resonant near-field fringe pattern. In order to record the interferogram, the nanospheres are deposited on a glass slide and their arrival positions are recorded via optical microscopy. We argue that the choice of silicon, due to its specific material characteristics, will yield reliable high-mass interference, unaffected by environmental decoherence, in a set-up that can be realized with present-day technology. Proposed experiment The proposed scheme is sketched in Fig. 1 . In the first stage of the experiment, a silicon particle is captured in an optical dipole trap by a lens system of numerical aperture 0.8 focusing a 1,550 nm laser to a waist of 860 nm (ref. 26 ); the interaction of nanoparticles with light is described further in Supplementary Note 1 . The trapping light is collected and used to determine the position of the particle [18] , which is feedback cooled over many trapping cycles to about T =20 mK of mean translational energy along the horizontal x -axis, implying a momentum uncertainty of about σ p / m =1.2 cm s −1 . A laser power of 55 mW results in a trap frequency of ν M =200 kHz and a position uncertainty σ x <10 nm; see Supplementary Note 2 . The trap thus serves as a nearly point-like matter-wave source for diffraction. 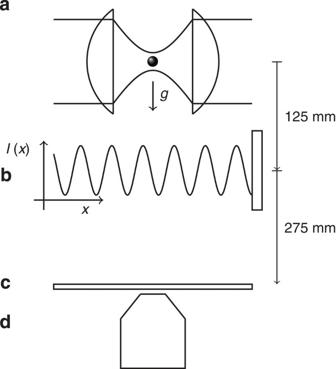Figure 1: Schematic of the proposed experiment. (a) Laser light at 1,550 nm creates a harmonic trap for single-silicon nanospheres. After feedback cooling to 20 mK, the particle is released and falls for 125 mm, where it passes a phase grating (b) provided by a retro-reflected nanosecond pulse at 355 nm. 275 mm further down the particle is adsorbed on a glass slide (c), where the arrival position is recorded with 100 nm accuracy via optical microscopy (d). Figure 1: Schematic of the proposed experiment. ( a ) Laser light at 1,550 nm creates a harmonic trap for single-silicon nanospheres. After feedback cooling to 20 mK, the particle is released and falls for 125 mm, where it passes a phase grating ( b ) provided by a retro-reflected nanosecond pulse at 355 nm. 275 mm further down the particle is adsorbed on a glass slide ( c ), where the arrival position is recorded with 100 nm accuracy via optical microscopy ( d ). Full size image After feedback cooling, the particle is released from the trap and falls for t 1 =160 ms before it is illuminated by a frequency-trippled Nd:YAG laser pulse at 355 nm with a pulse length of 10 ns and an energy E G ≤500 μJ. The pulse is retro-reflected by a mirror to form a standing-wave phase grating with period d = λ G /2, which diffracts the particle by modulating the matter-wave phase through the dipole interaction. The Talbot time, which sets the scale for near-field interference [3] , is thus given by t T = md 2 / h ≈80 ms. The laser beam must be expanded such that the waist is larger than the uncertainty in position σ p t 1 / m ≈2 mm accrued during free flight. Moreover, the orientation of the grating must be angularly stable to less than micro-radians to avoid blurring of the interferogram due to acceleration of the particle under gravity, and positionally stable to within 30 nm relative to the initial particle position; see Supplementary Note 3 . After the grating, the particle undergoes free fall for t 2 =126 ms, forming an interference pattern when it arrives on the glass slide. The arrival position can be detected by absorption imaging with visible light. Fitting to the known point-spread function of the imaging system permits 100 nm positional accuracy [27] ; see Supplementary Note 4 . The density pattern depicted in Fig. 2a is predicted to appear after many runs of the experiment. In the following, we discuss the theoretical description of the interference effect and the experimental constraints. 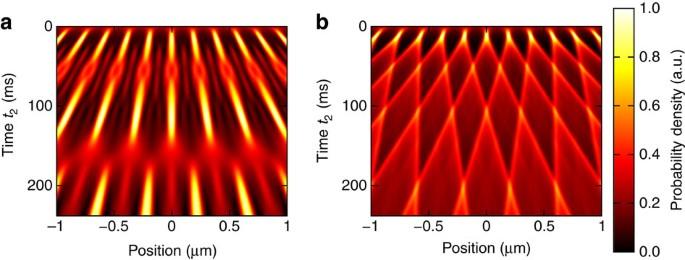Figure 2: Simulated fringe patterns below the grating. (a) Quantum and (b) classical probability densities at different timest2after the grating pulse. We assume the width of the trap state to beσx=10 nm and a time of flight to the grating oft1=160 ms; the grating has the periodd=177 nm with the maximal phase modulation set toφ0=π. The interference pattern is detected aftert2=126 ms in the set-up ofFig. 1. Quantum mechanics then predicts high-contrast fringes, which cannot be explained classically. Figure 2: Simulated fringe patterns below the grating. ( a ) Quantum and ( b ) classical probability densities at different times t 2 after the grating pulse. We assume the width of the trap state to be σ x =10 nm and a time of flight to the grating of t 1 =160 ms; the grating has the period d =177 nm with the maximal phase modulation set to φ 0 = π . The interference pattern is detected after t 2 =126 ms in the set-up of Fig. 1 . Quantum mechanics then predicts high-contrast fringes, which cannot be explained classically. Full size image Theoretical model Our starting point for evaluating the interference effect is the trapped thermal state of motion, a Gaussian mixture with standard deviations and . The particle will be illuminated by a uniform standing-wave pulse oriented along the horizontal x -axis (see Fig. 1 ), so that the y - and z -motion can be ignored. The near-field diffraction effect including all relevant decoherence mechanisms is best captured in a quantum phase-space description [28] . For the present purposes it is most useful to work with the characteristic function representation χ ( s , q ), that is, the Fourier transform of the Wigner function [29] of a given quantum state ρ . Here, we summarize the detailed derivation given in Supplementary Methods . The initial Gaussian state, first evolves freely for a time t 1 , χ 1 ( s , q )= χ 0 ( s − qt 1 / m , q ), before it is illuminated by the optical grating pulse of period d . Given an almost point-like initial spread σ x / d ≪ 1, the matter waves must evolve for at least the Talbot time t T to ensure that they are delocalized over adjacent grating nodes in order to be able to interfere. The initial momentum, on the other hand, is spread over many grating momenta, σ p d / h >>1, so that the time-evolved state extends over many grating periods. That is, if particles are only detected in a finite detection window around the centre of the distribution in the end, we can neglect the Gaussian density profile by writing The particle interacts with the standing-wave pulse through its optical polarizability , determined by the particle radius R and its complex refractive index n Si at the grating wavelength λ G =2 d . In the limit of short pulse durations τ , this imprints the phase φ ( x )= φ 0 cos 2 ( πx / d ) on the matter-wave state [15] , where φ 0 =2Re( α ) E G / ħcε 0 a G depends on the energy E G and spot area a G of the pulse. The characteristic function transforms as , where the B n are Talbot coefficients, given in terms of Bessel functions [30] , Incoherent effects due to absorption or scattering of laser photons are negligible for the nanoparticles considered here ( Supplementary Methods ); nevertheless, our numerical simulations include both effects. The final density distribution w ( x )=‹ x | ρ | x ›, that is, the probability to find the particle at position x after another free time evolution by t 2 , then takes the form It describes a periodic fringe pattern oscillating at the geometrically magnified grating period D = d ( t 1 + t 2 )/ t 1 (ref. 25 ). The fringe amplitudes, given by the Talbot coefficients (3), are diminished the larger the spread σ x of the initial state (1). An exemplary density pattern (4) is plotted in Fig. 2a for varying time t 2 . The simulation was performed for 10 6 AMU silicon particles, assuming realistic experimental parameters and including the influence of environmental decoherence. It shows pronounced interference fringes with visibilities of up to 75%. The pattern in Fig. 2b is the result of a classical simulation assuming that the particles are moving on ballistic trajectories. A lensing effect due to the strong dipole forces exerted by the standing-wave field is here responsible for the density modulation. This classical result is obtained simply by replacing sin πξ by πξ in expression (3) for the grating coefficients [30] . The clear difference between the quantum and the classical pattern is captured by the sinusoidal fringe visibility, the ratio between the amplitude and the offset of a sine curve of period D fitted to the density pattern (4): As shown in Fig. 3 , the classical and the quantum prediction differ significantly: the classical theory predicts many regions of low contrast as a function of φ 0 , whereas the quantum prediction exhibits a slow φ 0 dependence. The highest quantum visibility amounts to 83% at φ 0 =1.4 π . 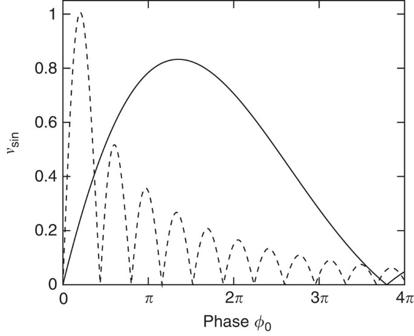Figure 3: Expected quantum (solid) and classical (dashed) sinusoidal visibilities as a function of the phase-modulation parameterφ0. This dependence on the pulse energy illustrates clearly the difference between the predictions. Figure 3: Expected quantum (solid) and classical (dashed) sinusoidal visibilities as a function of the phase-modulation parameter φ 0 . This dependence on the pulse energy illustrates clearly the difference between the predictions. Full size image Accounting for decoherence A realistic assessment of the proposed scheme must also include the influence of collisional and thermal decoherence [28] . This is incorporated into (4) by multiplying each Fourier component with a reduction factor of the form where Γ gives the rate and f ( x ) determines the spatial resolution of decoherence events of a certain class. In our simulation we accounted for collisions with residual gas particles, scattering and absorption of blackbody photons, and thermal emission of radiation using a realistic microscopic description. Each process contributes another factor R n listed in the Supplementary Methods ; the rate of thermal emission depends on time since the particle loses internal energy and cools during flight. Experimental constraints As a major concern for the successful implementation of the experiment, environmental decoherence must be kept sufficiently low. According to our simulations, collisional decoherence can be essentially avoided at ultra-high vacuum pressures of 10 −10 mbar. Radiative decoherence is suppressed by choosing silicon spheres because they are essentially transparent at typical wavelengths of room temperature blackbody radiation. The thermal emission of photons is determined by the internal temperature of the nanospheres, which is set in the trapping stage of the experiment. A trapping intensity of 90 mW μm −2 leads to an initial heating rate ∂ t T int =200 K s −1 and an equilibrium temperature of 1,600 K. This high value is a consequence of the low blackbody emissivity of silicon [31] , implying that the particle does not lose heat efficiently while in the trap. Nevertheless, due to the high refractive index n Si =3.48 of silicon, the particle may be trapped for well in excess of a second before the temperature rises that high. This time corresponds to about 10 5 trap oscillations, a sufficient period to perform parametric feedback cooling of the motion to T =20 mK; see Supplementary Note 5 . The low emissivity of silicon is the essential advantage compared to other materials such as silica, for which much work in this field has been done [10] , [11] , [23] . We find that to perform this experiment with silica would require cryogenic cooling of both apparatus and nanoparticle to 100 K, whereas thermal decoherence of silicon becomes important only at internal temperatures in excess of 1,000 K. Moreover, the high refractive index of silicon compared to the value n SiO2 =1.44 of silica means that less optical power is required to trap the sphere and to monitor its position [24] . As an additional advantage, silicon absorbs strongly at optical frequencies, which simplifies the detection of the interferogram. In principle, this would also affect the interaction with the grating laser, since a particle at the anti-node of the grating absorbs on average n 0 =0.12 φ 0 photons. For a grating laser waist of 30 mm we anticipate a phase modulation of φ 0 / E G =50 rad mJ −1 and hence we can access φ 0 ≤4 π . The finite absorption of grating photons, which is included in the simulations, disturbs the interferogram little. We presented a viable scheme for high-mass nanoparticle interferometry, which employs only a single optical diffraction element and requires only moderate motional cooling. The set-up would operate in ultra-high vacuum at room temperature. It is limited to masses up to 10 6 AMU mainly by the growing Talbot time and free-fall distance [32] . Interferometry in a microgravity environment could pave the way to even higher masses [33] . Remarkably, with path separations of up to 150 nm and interrogation times of 300 ms, the presented scheme is already sensitive to alternative theories beyond the Schrödinger equation. The renowned collapse model of continuous spontaneous localization (CSL) [34] could be probed in its current formulation [4] . In fact, a successful demonstration of interference with a visibility exceeding 42% would bound the localization rate to λ CSL <1.4 × 10 −11 Hz, a value at the lower end of recent estimates for this parameter [35] , [36] ; see Supplementary Discussion . Such a superposition experiment can be associated with a macroscopicity value of μ =18 (ref. 37 ), substantially exceeding that of every present-day matter-wave experiment and comparing well with the most ambitious micromirror superposition proposals [9] . How to cite this article: Bateman, J. et al . Near-field interferometry of a free-falling nanoparticle from a point-like source. Nat. Commun. 5:4788 doi: 10.1038/ncomms5788 (2014).